Numerical chromosomal instability mediates susceptibility to radiation treatment The exquisite sensitivity of mitotic cancer cells to ionizing radiation (IR) underlies an important rationale for the widely used fractionated radiation therapy. However, the mechanism for this cell cycle-dependent vulnerability is unknown. Here we show that treatment with IR leads to mitotic chromosome segregation errors in vivo and long-lasting aneuploidy in tumour-derived cell lines. These mitotic errors generate an abundance of micronuclei that predispose chromosomes to subsequent catastrophic pulverization thereby independently amplifying radiation-induced genome damage. Experimentally suppressing whole-chromosome missegregation reduces downstream chromosomal defects and significantly increases the viability of irradiated mitotic cells. Further, orthotopically transplanted human glioblastoma tumours in which chromosome missegregation rates have been reduced are rendered markedly more resistant to IR, exhibiting diminished markers of cell death in response to treatment. This work identifies a novel mitotic pathway for radiation-induced genome damage, which occurs outside of the primary nucleus and augments chromosomal breaks. This relationship between radiation treatment and whole-chromosome missegregation can be exploited to modulate therapeutic response in a clinically relevant manner. Radiation therapy is an integral modality in cancer treatment [1] . The lethal effect of ionizing radiation (IR) lies in its ability to cause widespread genomic damage primarily in the form of DNA double-strand breaks (DSBs). Each gray (Gy) of IR has been proposed to directly induce ~35 DNA DSBs per cell [2] . This overwhelming damage generally overcomes the ability of tumour cells to repair DSBs, leading to reduction in cellular viability and cell death. DNA damage produced by IR can be repaired through homologous recombination and non-homologous end joining. Non-homologous end joining can also erroneously join DSB ends of genomic DNA, which can lead to chromosomal translocations, acentric chromatin fragments as well as dicentric chromosomes [3] . Acentric chromatin fragments exhibit a high likelihood of missegregation during the subsequent mitosis, as they are incapable of establishing canonical attachment to spindle microtubules at the kinetochores. Alternatively, dicentric chromatin often leads to the formation of chromatin bridges where each centromere is attached to microtubules emanating from opposite spindle poles. Forces exerted by the mitotic spindle break chromatin bridges in a process termed the breakage-fusion-bridge cycle [4] . This cycle can also be initiated by telomere dysfunction and replication stress. It is thus clear that DNA breaks generated by IR in dividing cells can directly lead to structural chromosomal instability (s-CIN), whose mitotic hallmarks are chromatin bridges and acentric chromatin fragments [5] . Another form of genome instability, present in the majority of solid tumours, is numerical (or whole-) chromosomal instability (w-CIN) [6] . w-CIN primarily arises from errors in whole-chromosome segregation during mitosis [5] , [7] and it generates widespread aneuploidy in tumour cells [8] . A phenotypic hallmark of w-CIN, both in cell culture and human tumour samples, is the presence of chromosomes that lag in the middle of the mitotic spindle during anaphase [8] , [9] , [10] . These lagging chromosomes can directly lead to chromosome missegregation and aneuploidy. w-CIN does not exist in isolation, as it was recently shown that lagging chromosomes can also undergo severe structural damage by generating whole-chromosome-containing micronuclei [11] . These micronuclei are defective in DNA replication and repair and possess a faulty nuclear envelope [12] , leading to the pulverization of their enclosed chromosomes. Thus, w-CIN can in turn lead to s-CIN. Given the interrelatedness of w-CIN and s-CIN, we asked whether IR could directly generate numerical chromosomal abnormalities. Experimental and clinical evidence suggest that, in addition to direct DNA breaks, IR can lead to changes in chromosome number [13] , [14] , [15] , [16] . Furthermore, we recently demonstrated that activation of the DNA damage response pathway during mitosis, using IR or Doxorubicin, directly leads to the formation of lagging chromosomes during anaphase [17] . This suggests that IR has the potential to generate both w-CIN and s-CIN in a context-dependent manner. The sensitivity of cells to IR is not only dependent on the amount of DNA damage that immediately results from IR exposure, but on pre-existing damage or the inability to repair this damage are also important determinants of cellular viability [1] . In the clinical setting, the relationship between s-CIN and IR has long been recognized [1] , [18] , whereby genetically unstable tumours with intrinsically elevated rates of s-CIN or decreased DNA repair ability are more likely to respond to radiation treatment. Accordingly, many chemotherapeutic agents that sensitize tumours to IR act by either promoting DNA damage or impairing DNA repair [19] . On the other hand, the role of w-CIN in mediating sensitivity to IR is much less understood. This is particularly relevant given that mitosis has long been recognized as the most radiosensitive phase of the cell cycle [20] , [21] , thus offering a potentially important therapeutic target. Along these lines, we recently found that, in patients diagnosed with rectal adenocarcinoma, elevated pre-treatment rates of chromosome segregation errors forebode superior response to chemoradiation therapy [22] . This suggests that pre-existing defects related to w-CIN that manifest as lagging chromosomes may also play a role in determining sensitivity to IR. Here we use high-resolution immunofluorescence microscopy and xenograft mouse models to directly examine the consequences of IR exposure during mitosis on chromosome segregation and structural integrity as well as cellular karyotypes. We then experimentally reduce mitotic whole-chromosome missegregation rates to dissect the role of w-CIN on cellular viability in vitro and i n vivo in response to radiation treatment. IR induces w-CIN in vitro We recently showed that IR exposure during mitosis directly induces chromosome segregation errors in a dose-dependent manner [17] . Herein, we examined three human cell lines derived from normal human retinal epithelium (RPE1), colorectal cancer (HCT116) or glioma (U251). These cells were either near-diploid and chromosomally stable (RPE and HCT116) or aneuploid and chromosomally unstable (U251). RPE1 and HCT116 had an intact p53-signalling pathway [23] , whereas U251 contain defective p53 signalling [24] . Cells were first exposed to IR and examined 25 min later for signs of chromosome segregation during anaphase. This provided sufficient time for many of the cells that were in mitosis during DNA damage induction to enter anaphase, but not sufficient time for cells that were in G2 to proceed through to anaphase [25] . We used high-resolution fluorescence microscopy to examine the various types of chromosome segregation errors during anaphase and found that IR exposure led to a significant increase in anaphase spindles with lagging chromosomes, acentric chromatin fragments, or both ( Fig. 1a,b ). These lagging chromosomes were phenotypically similar to those naturally occurring in chromosomally unstable cancer cells in that they contained centromere staining and maintained attachments to microtubules emanating from opposite spindle poles ( Supplementary Fig. 1a ). Lagging chromosomes observed after IR exposure exhibited similar levels of staining of γ-H2AX, a marker of DNA DSBs, compared with the remaining chromosomes ( Supplementary Fig. 1b ). Furthermore, in these cells, we did not observe a significant increase in spindles with chromatin bridges ( Fig. 1a,b ). 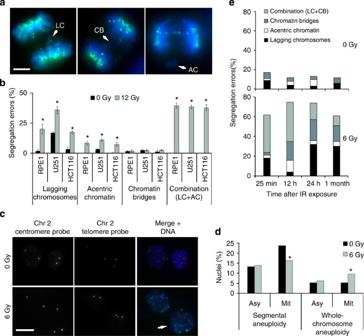Figure 1: Ionizing radiation (IR) leads to numerical chromosomal instability. (a) Examples of U251 cells fixed 25 min after exposure to 12 Gy and exhibiting lagging chromosomes (LC), chromatin bridges (CB), acentric chromatin (AC) or a combination (LC+AC). Cells were stained for centromeres (green) and DNA (blue). Scale bar, 5 μm (b) Percentage of chromosome missegregation in anaphase spindles of RPE1, HCT116 and U251 cells as a function of IR dose. Bars represents mean±s.e.m.,n=150 cells, three experiments, *P<0.01, two-tailedt-test. (c) Examples of HCT116 nuclei stained for DNA (blue), centromere (red) and telomere (green) probes for human chromosome 2. White arrow denotes an aneuploid nucleus containing three copies of chromosome 2. Scale bar, 10 μm. (d) Per cent HCT116 nuclei containing whole-chromosome and segmental aneuploidy for chromosome 2.n=300 cells, *P<0.05. (e) Percentage of chromosome missegregation in anaphase spindles of HCT116p53−/−cells exposed to 0 Gy (top) or 6 Gy (bottom) as a function of time after irradiation (mo, months). Figure 1: Ionizing radiation (IR) leads to numerical chromosomal instability. ( a ) Examples of U251 cells fixed 25 min after exposure to 12 Gy and exhibiting lagging chromosomes (LC), chromatin bridges (CB), acentric chromatin (AC) or a combination (LC+AC). Cells were stained for centromeres (green) and DNA (blue). Scale bar, 5 μm ( b ) Percentage of chromosome missegregation in anaphase spindles of RPE1, HCT116 and U251 cells as a function of IR dose. Bars represents mean±s.e.m., n =150 cells, three experiments, * P <0.01, two-tailed t -test. ( c ) Examples of HCT116 nuclei stained for DNA (blue), centromere (red) and telomere (green) probes for human chromosome 2. White arrow denotes an aneuploid nucleus containing three copies of chromosome 2. Scale bar, 10 μm. ( d ) Per cent HCT116 nuclei containing whole-chromosome and segmental aneuploidy for chromosome 2. n =300 cells, * P <0.05. ( e ) Percentage of chromosome missegregation in anaphase spindles of HCT116 p53 −/− cells exposed to 0 Gy (top) or 6 Gy (bottom) as a function of time after irradiation (mo, months). Full size image To further assess the consequences of IR exposure, we exposed cells to 6 Gy and performed fluorescence in situ hybridization (FISH) using centromere and telomere probes for chromosome 2 on irradiated nuclei 1 h later ( Fig. 1c ). Exposure of non-synchronized cells to IR did not result in significant short-term change in chromosome number. Yet when we enriched for mitotic cells using a mitotic shake-off method, IR led to approximately twofold increase in aneuploidy as evidenced by balanced changes in both centromere and telomere probes specific to human chromosome 2 ( Fig. 1d ). We then asked whether the frequency and types of chromosome segregation errors were dependent on the time interval between IR exposure and the analysis of anaphase chromosome segregation. To address this, we assessed chromosome segregation errors in HCT116 p53 −/− at 25 min, 12 h, 24 h, and 1 month after exposure to 6 Gy of IR. These cells were homozygously deleted for the tumour suppressor, p53 , to allow for the proliferation of aneuploid cells [23] should they emerge. Anaphase spindles examined 25 min after irradiation exhibited similar chromosome missegregation profiles compared with p53-competent HCT116 cells 25 min after IR exposure ( Fig. 1e ). However, 12 h after irradiation there was a significant increase in chromatin bridges and acentric chromatin fragments but not lagging chromosomes ( Fig. 1e ). Interestingly, anaphase spindles examined 24 h or up to 1 month after IR exposure revealed a significant increase in both lagging chromosomes and chromatin bridges ( Fig. 1e ). This suggests that chromosome segregation errors in response to IR exposure are time dependent; lagging chromosomes peak shortly (25 min) after IR exposure, whereas chromatin bridges peak 12 h later. Importantly, long-term examination of irradiated cells shows persistence of lagging chromosomes and chromatin bridges, the hallmarks of w-CIN and s-CIN, respectively. IR induces w-CIN in vivo To determine whether IR can directly perturb the process of chromosome segregation in vivo , we made use of tumour-forming HCT116 p53 −/− cells that normally exhibit low rates of chromosomes missegregation and are thus considered chromosomally stable and near-diploid [23] . We subcutaneously injected HCT116 p53 −/− into nude mice and exposed transplanted tumours to 10 Gy followed by formalin-fixation 25 min later to focus on the effects of radiation on mitotic cells ( Fig. 2a,b ). Tumours exposed to 10 Gy of IR exhibited significantly higher rates of chromosome segregation errors during anaphase compared with control, non-irradiated, tumours ( Fig. 2c ). In tumours from irradiated animals, haematoxylin-stained chromatin was frequently visible in the central spindle during anaphase ( Fig. 2b , and insets). This chromatin often contained a central constriction reminiscent of centromeric DNA suggesting that this chromatin encompassed whole chromosomes. However, experimental limitations preclude us from resolving lagging chromosomes from acentric chromatin fragments with absolute certainty in fixed tumour tissues. 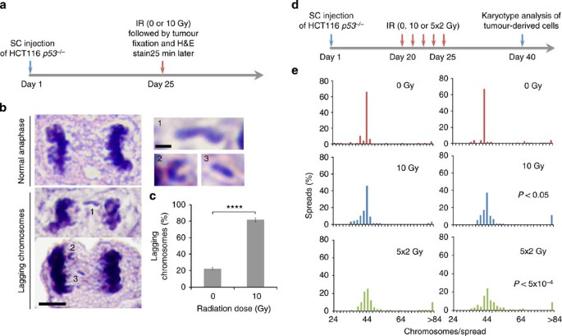Figure 2: Ionizing radiation (IR) induces chromosome segregation errorsin vivo. (a) Schema for experiments depicted inb,c. Gy, gray; H&E, haematoxylin and eosin; SC, sub-cutaneous. (b) Example of H&E-stained SC-HCT116p53−/−xenografts showing normal anaphase and anaphase cells containing lagging chromosomes. Scale bar, 5 μm, inset bar ,1 μm. (c) Percentage of anaphase cells exhibiting lagging chromosomes in SC-HCT116p53−/−xenografts as a function of radiation dose. Bars represent mean±s.d.,n=4 mice; ****P<0.0001, two-tailedt-test. (d) Schema for experiments depicted ine. (e) Karyotype distribution of cells derived from six SC-HCT116p53−/−xenografts, each histogram represents a 100 spreads derived from a single tumour, two-tailedt-test. Figure 2: Ionizing radiation (IR) induces chromosome segregation errors in vivo . ( a ) Schema for experiments depicted in b , c . Gy, gray; H&E, haematoxylin and eosin; SC, sub-cutaneous. ( b ) Example of H&E-stained SC-HCT116 p53 −/− xenografts showing normal anaphase and anaphase cells containing lagging chromosomes. Scale bar, 5 μm, inset bar ,1 μm. ( c ) Percentage of anaphase cells exhibiting lagging chromosomes in SC-HCT116 p53 −/− xenografts as a function of radiation dose. Bars represent mean±s.d., n =4 mice; **** P <0.0001, two-tailed t -test. ( d ) Schema for experiments depicted in e . ( e ) Karyotype distribution of cells derived from six SC-HCT116 p53 −/− xenografts, each histogram represents a 100 spreads derived from a single tumour, two-tailed t -test. Full size image We next exposed HCT116 p53 −/− xenografts to varying doses of radiation (0 Gy, 10 Gy and five daily fractions of 2 Gy over 5 consecutive days). As mitotic cells represent a minority of the tumour cell population at any given time, the latter fractionated regimen (2 Gy × 5 days) aims at targeting an overall larger number of mitotic cells over consecutive days. We subsequently derived cells from irradiated tumours and passaged them in culture for an additional 15 days to obtain sufficient numbers of cells for karyotype analysis ( Fig. 2d ). Cells derived from non-irradiated tumours displayed mitotic spreads with near-diploid karyotypes. In contrast, mitotic spreads of cells derived from irradiated tumours showed significant deviations from the near-diploid modal chromosome number—particularly those exposed to five daily fractions ( Fig. 2e ). There was also a small increase in near-tetraploid cells, which appeared to have undergone a genome-doubling event ( Fig. 2e ). Extra-nuclear DNA damage in irradiated mitotic cells In addition to aneuploidy, lagging chromosomes can lead to downstream defects that culminate in structural chromosomal damage [11] . The physical separation of lagging chromosomes from the remaining faithfully segregating ones during anaphase can lead to their exclusion from the primary nucleus in the subsequent G1 phase of the cell cycle, forming micronuclei. The nuclear envelopes that form around these chromosomes are defective and exhibit error-prone DNA replication and repair, predisposing their enclosed chromosomes to catastrophic pulverization [11] , [12] . We examined RPE1 and U251 cells 12 h after IR exposure and found increased frequencies of whole-chromosome-containing micronuclei that positively stained for both DNA and centromeres ( Fig. 3a–c ). We then irradiated mitotic cells obtained by mitotic shake-off and examined chromosome spreads 24 h after irradiation to assay for chromosome pulverization in the subsequent mitosis as previously described [11] ( Fig. 3d ). In these spreads, the appearance of many small chromosome fragments and decondensed chromatin indicate the consequences of chromosome pulverization [11] ( Fig. 3e ). 12 Gy of IR to mitotic U251 cells led to a significant increase in the fraction of chromosome spreads displaying pulverized chromosomes ( Fig. 3f ). 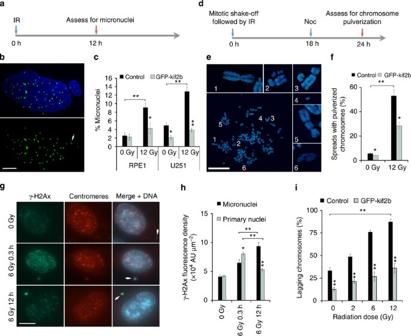Figure 3: IR-induced chromosome segregation errors lead to widespread chromosomal damage. (a) Experimental schema for assessing the generation of IR-induced micronuclei. (b) Example image of a U251 cell containing a micronucleus stained for centromeres (green) and DNA (blue), scale bar, 5 μm. (c) Percentage of RPE1 and U251 cells containing micronuclei as a function of IR dose. Bars represents mean±s.e.m.,n=266–824 cells, three experiments, *P<0.05, **P<0.001, two-tailedt-test. (d) Experimental schema for assessing the generation of IR-induced chromosome pulverization. (e) Representative mitotic spread containing pulverized chromosomes from U251 cells irradiated with 12 Gy 24 h prior. Scale bar, 20 μm, which show a normal appearing chromosome (1), chromosome fragments (2–4), a dicentric chromosome (5) and uncondensed chromatin (6). (f) Percentage of mitotic spreads from containing pulverized chromosomes from control and U251 cells expressing GFP-Kif2b. Bars represent mean±s.e.m.;n>450 mitotic spreads, three experiments, *P<0.05, **P<0.001, two-tailedt-test. (g) Examples of U251 cells, exposed to 0 Gy, 6 Gy and fixed either 0.3 or 12 h later, containing micronuclei that encompass whole chromosomes (arrows) as evidenced by centromere staining (red) that were also stained for γ-H2AX (green) and DNA (blue). Scale bar, 5 μm (h) γ-H2AX fluorescence intensity in primary nuclei and micronuclei in U251 cells exposed to 0 and 12 Gy stained 0.3 or 12 h after irradiation. AU, arbitrary units; bars represent mean±s.e.m.;n>30 cells, three experiments, *P<0.05, **P<0.001, two-tailedt-test. (i) Percentage of anaphase spindles containing lagging chromosomes as a function of IR dose, in control and GFP-Kif2b-overexpressing U251 cells. Bars represents mean±s.e.m.,n=150 cells, three experiments, **P<0.001, two-tailedt-test. Figure 3: IR-induced chromosome segregation errors lead to widespread chromosomal damage. ( a ) Experimental schema for assessing the generation of IR-induced micronuclei. ( b ) Example image of a U251 cell containing a micronucleus stained for centromeres (green) and DNA (blue), scale bar, 5 μm. ( c ) Percentage of RPE1 and U251 cells containing micronuclei as a function of IR dose. Bars represents mean±s.e.m., n =266–824 cells, three experiments, * P <0.05, ** P <0.001, two-tailed t -test. ( d ) Experimental schema for assessing the generation of IR-induced chromosome pulverization. ( e ) Representative mitotic spread containing pulverized chromosomes from U251 cells irradiated with 12 Gy 24 h prior. Scale bar, 20 μm, which show a normal appearing chromosome (1), chromosome fragments (2–4), a dicentric chromosome (5) and uncondensed chromatin (6). ( f ) Percentage of mitotic spreads from containing pulverized chromosomes from control and U251 cells expressing GFP-Kif2b. Bars represent mean±s.e.m. ; n >450 mitotic spreads, three experiments, * P <0.05, ** P <0.001, two-tailed t -test. ( g ) Examples of U251 cells, exposed to 0 Gy, 6 Gy and fixed either 0.3 or 12 h later, containing micronuclei that encompass whole chromosomes (arrows) as evidenced by centromere staining (red) that were also stained for γ-H2AX (green) and DNA (blue). Scale bar, 5 μm ( h ) γ-H2AX fluorescence intensity in primary nuclei and micronuclei in U251 cells exposed to 0 and 12 Gy stained 0.3 or 12 h after irradiation. AU, arbitrary units; bars represent mean±s.e.m. ; n >30 cells, three experiments, * P <0.05, ** P <0.001, two-tailed t -test. ( i ) Percentage of anaphase spindles containing lagging chromosomes as a function of IR dose, in control and GFP-Kif2b-overexpressing U251 cells. Bars represents mean±s.e.m., n =150 cells, three experiments, ** P <0.001, two-tailed t -test. Full size image To assess the relative levels of DNA damage in the micronuclei compared with the primary nuclei, we measured the fluorescence density of γ-H2AX. Without irradiation both primary nuclei and micronuclei had equivalent densities of γ-H2AX fluorescence, which then significantly increased 25 min after IR exposure. As expected, γ-H2AX density in primary nuclei was significantly lower 12 h after IR exposure compared with 25 min, congruent with DNA repair activity ( Fig. 3g,h ). Conversely, γ-H2AX density in micronuclei was significantly increased at 12 h as compared with 25 min after IR exposure ( Fig. 3g,h ). This suggests that micronuclei are not only defective in DNA repair but can actively generate additional DNA damage. This additional damage is likely the consequence of faulty attempts at DNA repair [11] and defective micronuclei nuclear envelope structures [12] . Therefore, by inducing mitotic errors, IR can lead to amplifications of structural chromosomal defects that predominantly occur outside of the primary nucleus (extra-nuclear). Unlike DNA damage caused directly by IR, these defects are precipitated many hours after IR exposure. To corroborate that this extra-nuclear chromosomal damage occurs as a result of mitotic chromosome segregation errors, we measured lagging chromosomes 25 min after irradiation in U251 cells overexpressing GFP-Kif2b ( Fig. 3i and Supplementary Fig. 1c ). Kif2b is a microtubule-depolymerizing kinesin-13 protein that specifically corrects erroneous microtubule attachments to chromosomes [26] , [27] . Its overexpression was shown to selectively reduce whole-chromosome segregation errors and suppression of w-CIN in clonogenic assays in many cancer cell lines, including U251 cells [5] , [26] . It does so by reducing the stability of microtubule attachments to chromosomes at kinetochores, which are frequently elevated in chromosomally unstable cancer cell lines [28] . U251 cells overexpressing GFP-Kif2b displayed greater than twofold reduction in chromosome segregation errors during anaphase compared with control U251 cells ( Fig. 3i ) as well as fewer chromosome segregation errors during anaphase after IR exposure ( Fig. 3i ). In similar experiments, we found that GFP-Kif2b overexpression reduced the frequency of IR-induced lagging chromosomes in otherwise chromosomally stable RPE1 cells [17] . Accordingly, its overexpression also led to significant reductions in the frequency of cells containing micronuclei in both RPE1 and U251 cells ( Fig. 3c ). We then examined mitotic spreads, 24 h after exposure of mitotic cells to IR, for downstream chromosomal breaks known to result from micronuclei. GFP-Kif2b overexpression significantly reduced the incidence of spreads with pulverized chromosomes ( Fig. 3f ). This was not a complete suppression suggesting that chromosome pulverization in response to IR may also occur through alternative pathways unrelated to lagging chromosomes. To ensure that GFP-Kif2b overexpression did not alter the formation of direct DSBs in irradiated cells or the influence their ability to repair these breaks in primary nuclei, we measured relative γ-H2AX fluorescence intensity in irradiated mitotic cells and found no difference between control and GFP-Kif2b-overexpressing cells ( Fig. 4a ). Furthermore, we compared the average number of γ-H2AX foci in the primary nuclei 20 min and 12 h after IR exposure and found no significant difference between control and GFP-Kif2b-overexpressing cells ( Fig. 4b,c ). As expected, there was an approximately threefold decrease in the number of γ-H2AX foci 12 h following irradiation in both conditions, owing to DNA DSB repair activity ( Fig. 4b,c ). Thus, suppression of mitotic errors reduces extra-nuclear chromosomal defects without significantly altering the incidence of DNA DSBs in the primary nucleus or the rate at which they are repaired. 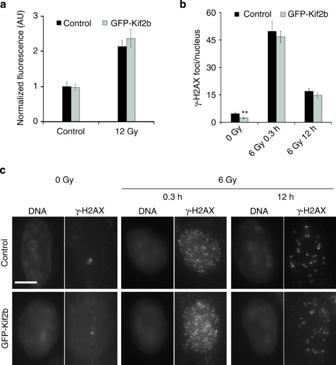Figure 4: Kif2b overexpression does not alter IR-induced DNA breaks or repair. (a) Normalized fluorescence intensity of γ-H2AX staining during mitosis in control and GFP-Kif2b-overexpressing U251 cells. Bars represent mean±s.e.m. (b) The average number of γ-H2AX foci per nucleus as a function of IR dose 20 min and 12 h after IR exposure of control and GFP-Kif2b-overexpressing U251 cells. Bars represent mean±s.e.m.,n=52–151 cells; **P<0.005, two-tailedt-test. (c) Examples of cells irradiated with 0 or 6 Gy stained for DNA (left) and γ-H2AX right. Scale bar, 5 μm. Figure 4: Kif2b overexpression does not alter IR-induced DNA breaks or repair. ( a ) Normalized fluorescence intensity of γ-H2AX staining during mitosis in control and GFP-Kif2b-overexpressing U251 cells. Bars represent mean±s.e.m. ( b ) The average number of γ-H2AX foci per nucleus as a function of IR dose 20 min and 12 h after IR exposure of control and GFP-Kif2b-overexpressing U251 cells. Bars represent mean±s.e.m., n =52–151 cells; ** P <0.005, two-tailed t -test. ( c ) Examples of cells irradiated with 0 or 6 Gy stained for DNA (left) and γ-H2AX right. Scale bar, 5 μm. Full size image w-CIN influences viability of irradiated mitotic cells Mitosis has long been recognized, for unclear reasons, as the most radiation sensitive phase of the cell cycle [1] , [20] , [21] . Having acquired the ability to selectively reduce chromosome segregation errors without influencing the canonical IR-induced DNA damage and repair within the primary nucleus, we could then ask whether whole-chromosome segregation errors might independently contribute towards the sensitivity of mitotic cells to IR. We assayed for the colony-forming ability of cells after exposure to increasing doses of IR, as previously described [1] , [29] . To focus on the potential effects of radiation on cells during mitosis, we enriched for mitotic cells using mitotic shake-off before irradiation and plating for colony growth. As expected, control U251 cells showed a dose-dependent reduction in the colony-forming capacity in response to radiation ( Fig. 5a ). Strikingly, GFP-Kif2b overexpression led to significant increase in the viability after irradiation, whereby at 12 Gy of IR, these cells were ~20-fold more resistant compared with control cells ( Fig. 5a ). Similarly, GFP-Kif2b overexpression led to increased viability in RPE1 cells albeit to a lesser extent ( Supplementary Fig. 2a ). Importantly, GFP-Kif2b overexpression did not alter the growth rate of U251 cells in culture or did it significantly influence their karyotypic distribution or modal chromosome numbers ( Supplementary Fig. 2b,c ). Overexpression of GFP-MCAK, a second kinesin-13 protein also known to suppress w-CIN in a slightly different manner [26] , led to a similar increase in clonogenic viability of mitotic cells ( Fig. 5a and Supplementary Fig. 1c ). Overexpression of either GFP alone or the third microtubule-depolymerizing kinesin-13 paralogue, GFP-Kif2a, which does not reduce chromosome segregation errors during mitosis [26] , did not alter the clonogenic potential of irradiated cells compared with control ( Fig. 5a , Supplementary Fig. 1c ). Interestingly, when we irradiated U251 cells as a non-synchronized population that contains only a small fraction of mitotic cells, overexpression of GFP-Kif2b did not influence the colony-forming ability ( Fig. 5b ). Collectively, these results suggest that chromosome segregation errors impact the viability of irradiated mitotic cells as the selective suppression of these errors through destabilization of kinetochore-microtubule stability leads to significant increase in mitotic cell resistance to IR. 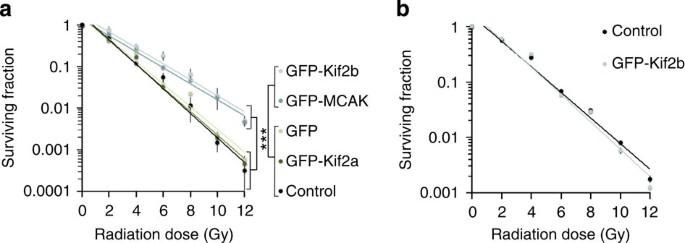Figure 5: Chromosome segregation errors alter the viability of irradiated mitotic cells. Surviving fraction of irradiated mitotically enriched (a) and non-synchronized (b) U251 cells as well as cells overexpressing GFP, GFP-Kif2a, GFP-MCAK or GFP-Kif2b. Circles denote mean±s.e.m.,n=3 experiments, ***P<0.005, two-tailedt-test. Figure 5: Chromosome segregation errors alter the viability of irradiated mitotic cells. Surviving fraction of irradiated mitotically enriched ( a ) and non-synchronized ( b ) U251 cells as well as cells overexpressing GFP, GFP-Kif2a, GFP-MCAK or GFP-Kif2b. Circles denote mean±s.e.m., n =3 experiments, *** P <0.005, two-tailed t -test. Full size image Suppressing w-CIN leads to tumour radiation resistance To test the relationship between chromosome segregation errors and tumour response to radiation in vivo , we intracranially transplanted U251 cells expressing firefly luciferase and either GFP or GFP-Kif2b into athymic mice. Eighteen days after cell injection, we delivered six fractions of 4 Gy (24 Gy total) over a period of 13 days ( Fig. 6a ). This dose fractionation regimen aims at targeting the most sensitive subpopulation of tumour cells—which include those undergoing mitosis during IR exposure—over multiple days while allowing cell cycle redistribution in the interval between radiation doses [1] , [30] , [31] , [32] . Absolute bioluminescence values before the initiation of treatment increased at comparable rates in GFP- and GFP-Kif2b-overexpressing tumours suggesting similar tumour growth rates ( Supplementary Fig. 3 ). Tumours overexpressing only GFP showed a robust response to radiation treatment as judged by approximately tenfold reduction in luciferase signal at the end of the treatment course ( Fig. 6b–d ). In contrast, there was striking resistance to radiation treatment in tumours derived from cells overexpressing GFP-Kif2b ( Fig. 6b–d ). This difference could not be accounted for by a proliferative disparity between GFP- and GFP-Kif2b-overexpressing tumours as both exhibited similar mitotic indices as well as equivalent proportions of cells that positively stained for the proliferation marker, Ki67 ( Fig. 6e–g ). GFP- and GFP-Kif2b-expressing tumours also exhibited similar frequencies of multipolar mitoses known to occur after radiation exposure [33] ( Fig. 6h,i ). However, GFP-Kif2b-expressing tumours displayed decreased apoptosis as indicated by lower cleaved caspase 3 staining ( Fig. 6j,k ). Therefore, suppression of numerical chromosomal instability by altering kinetochore-microtubule attachment stability leads to significant radiation resistance likely by suppressing cell death resultant from excessive chromosomal damage. 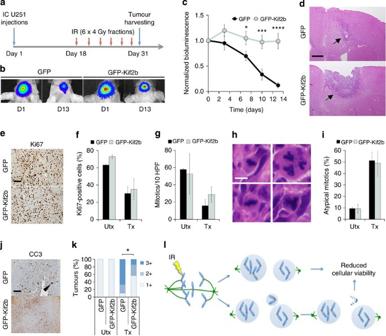Figure 6: Reducing chromosome segregation errors induces radiation resistancein vivo. (a) Experimental schema for assessingin vivotumour resistance; IC, intracranial. (b) Examples of bioluminescence images of mice harbouring IC GFP- and GFP-Kif2b-expressing tumours at day 0 (start of radiation treatment) and day 13 (end of radiation treatment). (c) Normalized bioluminescence signal overtime after initiation of IR treatment in IC GFP- and GFP-Kif2b-expressing U251 xenografts. Circles represent mean±s.e.m.,n=10 and 9 mice for GFP and GFP-Kif2b groups, respectively; *P<0.05, ***P<0.005, ****P<0.0001, two-tailedt-test. (d) Examples of haematoxylin and eosin-stained tumours expressing GFP or GFP-Kif2b, black arrows denote post-treatment tumours; scale bar, 500 μm. (e,f) Example of Ki67-stained specimens from irradiated tumours (e) and per cent Ki67-positive cells (f) in GFP- and GFP-Kif2b-expressing tumours. Bars represent mean±s.e.m.,n=2–4 mice (UTx) and 7–9 mice (Tx), 1,080–2,511 cells per tumour; scale bar, 100 μm. (g) Mitotic count (per 10 high-power fields) in treated (Tx) and untreated (UTx) GFP- and GFP-Kif2b-expressing U251 xenografts. Bars represent mean±s.e.m.,n=2–4 mice (UTx) and 7–9 mice (Tx). (h,i) Per cent of atypical mitotic cells (representative images depicted in h), in GFP- and GFP-Kif2b-expressing tumours. Bars represent mean±s.e.m.,n=2–4 mice (UTx) and 7–9 mice (Tx). Scale bar, 7 μm. (j,k) Example of cleaved caspase 3 (CC3)-stained specimens from irradiated tumours (j), and semi-quantitative CC3 staining score in tumours (k), 1+ (<0.5% CC3-positive cells), 2+ (0.5–3%), 3+ (>3%); *P=0.07,χ2-test,n=2–4 mice (UTx) and 7–9 mice (Tx), 1,080–2,511 cells per tumour; scale bar, 500 μm. (l) Schematic diagram linking IR to chromosome segregation errors and downstream chromosomal structural defects. Figure 6: Reducing chromosome segregation errors induces radiation resistance in vivo . ( a ) Experimental schema for assessing in vivo tumour resistance; IC, intracranial. ( b ) Examples of bioluminescence images of mice harbouring IC GFP- and GFP-Kif2b-expressing tumours at day 0 (start of radiation treatment) and day 13 (end of radiation treatment). ( c ) Normalized bioluminescence signal overtime after initiation of IR treatment in IC GFP- and GFP-Kif2b-expressing U251 xenografts. Circles represent mean±s.e.m., n =10 and 9 mice for GFP and GFP-Kif2b groups, respectively; * P <0.05, *** P <0.005, **** P <0.0001, two-tailed t -test. ( d ) Examples of haematoxylin and eosin-stained tumours expressing GFP or GFP-Kif2b, black arrows denote post-treatment tumours; scale bar, 500 μm. ( e , f ) Example of Ki67-stained specimens from irradiated tumours ( e ) and per cent Ki67-positive cells ( f ) in GFP- and GFP-Kif2b-expressing tumours. Bars represent mean±s.e.m., n =2–4 mice (UTx) and 7–9 mice (Tx), 1,080–2,511 cells per tumour; scale bar, 100 μm. ( g ) Mitotic count (per 10 high-power fields) in treated (Tx) and untreated (UTx) GFP- and GFP-Kif2b-expressing U251 xenografts. Bars represent mean±s.e.m., n =2–4 mice (UTx) and 7–9 mice (Tx). ( h , i ) Per cent of atypical mitotic cells (representative images depicted in h), in GFP- and GFP-Kif2b-expressing tumours. Bars represent mean±s.e.m., n =2–4 mice (UTx) and 7–9 mice (Tx). Scale bar, 7 μm. ( j , k ) Example of cleaved caspase 3 (CC3)-stained specimens from irradiated tumours ( j ), and semi-quantitative CC3 staining score in tumours ( k ), 1+ (<0.5% CC3-positive cells), 2+ (0.5–3%), 3+ (>3%); * P= 0.07, χ 2 -test, n =2–4 mice (UTx) and 7–9 mice (Tx), 1,080–2,511 cells per tumour; scale bar, 500 μm. ( l ) Schematic diagram linking IR to chromosome segregation errors and downstream chromosomal structural defects. Full size image Our work uncovers an additional layer of genome damage induced by IR, beyond direct DNA breaks, which occurs outside of the primary nucleus. We show that when IR is delivered to mitotic cells, it can directly lead to errors in whole-chromosome segregation, which subsequently leads to the formation of micronuclei and chromosome pulverization hours to days later ( Fig. 6l ). The type of missegregation errors in irradiated cells are dependent on the time lapsed after IR exposure. This is likely dependent on the phase of the cell cycle during which cells are irradiated. IR exposure during interphase (G1, S and G2) of the cell cycle would produce DSBs, which lead to acentric chromatin and chromatin bridges during the subsequent anaphase. This explains the prevalence of chromatin bridges and acentric chromatin 12 h after IR exposure ( Fig. 1b ). On the other hand, when cells are irradiated during mitosis this directly leads to the formation of lagging chromosomes. Interestingly, analysis of anaphase spindles 24 h, and up to 1 month, after IR exposure reveals chromosome missegregation patterns suggestive of both w-CIN and s-CIN. This mirrors recent work showing that w-CIN and s-CIN coexist in an interdependent manner [11] , [17] . This multilayered genomic damage represents a plausible explanation for the exquisite sensitivity of mitotic cells to IR [1] , [20] , [34] , whereby IR exposure during mitosis not only leads to direct DNA breaks but also to additional numerical and downstream structural chromosomal damage. This cell cycle-dependent sensitivity has been exploited in the way radiation treatment is delivered in clinical settings. A fundamental rational for dividing radiation treatment dose into small daily fractions is to enact lethal damage onto the sensitive subpopulation of tumour cells, including the mitotic subpopulation, while sparing toxicity to the surrounding normal tissue which typically contains fewer mitotic cells and is more adept at DNA repair [1] . Therefore, fractionated radiation therapy can maximize damage to mitotic cell population in otherwise non-synchronized tumours. The magnitude of the effect of Kif2b overexpression in vivo was surprising given the fact that most of the tumour cell population is not in M-phase. We postulate that some of this may be accounted for by the fractionation scheme with which we delivered radiation therapy. Second, when U251 cells are irradiated in vivo they exhibit increased rate of atypical mitoses ( Fig. 6h,i ). These spindle defects are likely caused by pre-mitotic damage as direct IR exposure during mitosis has not been shown to significantly alter spindle geometry [17] . The mechanism of how pre-mitotic irradiation induces spindle damage is poorly understood. Nonetheless, these atypical spindle geometries have been shown to lead to chromosome segregation errors [35] , [36] . Thus, it is conceivable that the effect of Kif2b overexpression in vivo extends beyond the directly irradiated mitotic tumour subpopulation whereby Kif2b suppresses w-CIN indirectly caused by defects in spindle geometry originating from pre-mitotic damage. This hypothesis is supported by the observation that DNA damage-induced cell death is enhanced by progression through mitosis [37] and we propose that this is partly due to numerical chromosomal aberration resulting from mitotic chromosome missegregation. The dependence of irradiated mitotic cell sensitivity on chromosome missegregation rates offers insight into recent findings where patients diagnosed with rectal adenocarcinoma with elevated pre-treatment chromosome segregation errors are more likely to respond to chemoradiation therapy [22] . Interestingly, in this patient cohort, there was a synergistic relationship in the predictive power between chromosome missegregation and levels of Mre11, a component of the MRN complex involved in the recognition and repair of DSBs [38] . Patients with elevated chromosome missegregation and reduced levels of Mre11 were significantly more likely to respond to chemoradiation therapy [22] . This suggests that increasing chromosome missegregation rates in mitosis may increase the therapeutic potency of IR particularly in the setting of decreased repair efficiency of DSBs. Such an approach may already be within clinical feasibility as several known chemotherapeutics can increase chromosome missegregation rates [23] , [39] , [40] , [41] . It can also be achieved more selectively by developing molecularly targeted inhibitors of the kinesin-13 proteins, Kif2b or MCAK. The severe structural damage caused by the effect of IR on mitotic cells has important consequences on the small subset of cells that survive radiation treatment. Chromosome pulverization has been postulated to represent a precursor to massive chromosomal rearrangements known as chromothripsis [42] . Our results suggest that pulverization is likely deleterious to cellular viability. In rare instances, however, these punctuated genomic alterations could lead to selective advantage and generate highly aggressive tumours [42] , which represent a rare but devastating late side-effect of radiation therapy [1] . Our work predicts that chromosome pulverization and subsequent chromothripsis would be a defining feature of radiation-induced secondary tumours. Cell culture and irradiation Cells were maintained at 37 °C in a 5% CO 2 atmosphere in DMEM (for U251) or McCoy’s medium (for HCT116) with 10% fetal bovine serum, 50 IU ml −1 penicillin and 50 μg ml −1 streptomycin. U251 cells were kindly provided from the laboratory of Mark A. Israel (Geisel School of Medicine at Dartmouth), HCT116 cells (both p53 +/+ and p53 −/− ) were kindly provided by the laboratory of Bert Vogelstein (Johns Hopkins University). For plasmid selection, cells were maintained in 0.5–1.0 mg ml −1 of G418 (geneticin). Cells were γ-irradiated using a 137 Cs-irradiator at a rate of 2.38 Gy min −1 or using external beam radiation at 6 MeV delivered by a linear accelerator according to safety rules of Dartmouth and University of California, San Francisco. Antibodies Tubulin-specific mAb DM1α (Sigma-Aldrich), anti-centromere antibody (CREST), anti-CC-3 antibody (Cell Signaling), anti-Ki67-antibody (Ventana), anti-γ-H2AX-antibody (Novus Biologicals), GFP-specific antibody (William Wickner). Antibodies were used at dilutions of 1:1,000 or 1:10,000 (for GFP-specific antibody). Immunofluorescence imaging Cells were fixed with 3.5% paraformaldehyde or methanol (−20 °C) for 15 min, washed with Tris-buffered saline with 5% bovine serum albumin (TBS-BSA) and 0.5% Triton X-100 for 5 min, and TBS-BSA for 5 min. Antibodies were diluted in TBS-BSA+0.1% Triton X-100 and coverslips incubated for 3 h at room temperature, then washed with TBS-BSA for 5 min. Secondary antibodies were diluted in TBS-BSA+0.1% Triton X-100 and coverslips incubated for 1 h at room temperature. Images were acquired with Orca-ER Hamamatsu cooled CCD camera mounted on an Eclipse TE 2000-E Nikon microscope. 0.2 μm optical sections in the z -axis were collected with a plan Apo × 60 1.4 numerical aperture oil immersion objective at room temperature. Iterative restoration was performed using Phylum Live software (Improvision). Quantification of γ-H2AX fluorescence levels were done using Phylum. Immunoblots Membranes were blocked with 0.5% milk in TBS+0.1% Tween for 1 h. Membranes were blotted at room temperature for 3 h with antibodies at 1:1,000. Secondary HRP-conjugated anti-mouse/rabbit (Bio-Rad) were used at 1:2,000. Images of uncropped immunoblots are depicted in Supplementary Fig. 4 . Fluorescence in situ hybridization HCT116 p53 −/− cells were treated with 100 μM monastrol or dimethylsulphoxide control for 8 h and then γ-irradiated. Immediately following irradiation, cells were washed with PBS twice and then recovered in fresh media for 1 h. For FISH analysis, cells were collected by trypsinization, briefly resuspended in 75 mM potassium chloride, fixed, washed twice in 3:1 methanol/acetic acid mix, dropped onto wet slides, air dried and stained with 4,6-diamidino-2-phenylindole. FISH was performed using both α-satellite and subtelomere probes specific for the centromeric and q arm telomeric regions of chromosomes 2, respectively (Cytocell). Cells were hybridized according to the manufacturer’s protocol, and chromosome signals in at least 300 nuclei were scored. In vivo xenograft HCT116 experiments Animal experiments were approved by Institutional Animal Cancer and Use Committee at UCSF, in accordance with institutional and national guidelines. 2–5 million HCT116 p53 −/− cells [43] were implanted subcutaneously into the flanks of CD1-Nude mice (4- to 6-week-old males supplied by the UCSF Breeding Core or Jackson Labs). Tumours were measured with calipers. Volume was calculated by the following formula: width 2 × length × 0.5. Tumours were exposed to gamma irradiation ( 137 Cs) at fractionated doses (5 consecutive days × 2 Gy) when tumours were ~300 mm 3 or at a single dose (1 day × 10 Gy) when tumours were ~800 mm 3 . Tumours were isolated and cultured or sectioned for immunohistochemistry. Clonogenic assays Cells were either trypsinized (for non-synchronized populations) or collected using mitotic shake-off (for mitotic population) serially diluted and irradiated in their native medium. Cells were then plated in 25-cm 2 T-flasks and clones were grown for 18 days. Clones were stained with Crystal violet and colonies were counted when they reached an approximate size of ~50 cells per clone [29] . Relative viability was determined based on the 0-Gy dose. Automated counting of γ-H2AX foci Cell Profiler 2.0 (Broad Institute) [44] was used to segment nuclei and for automated counting of foci using the examplesspeckles.cp pipeline. Nuclei were segmented based on their shape and signal intensity, foci were identified based on their intensity and their diameter. Intensity threshold spanned 2.5–100%. In vivo orthotopic U251 experiments Mouse experiments were approved by and performed according to the guidelines of the Institutional Animal Cancer and Use Committee at UCSF. U251-GFP-Kif2b and U251-GFP cells were modified using lentivirus expressing firefly luciferase. Dissociated cells were resuspended in ice-cold DME H-21 medium without supplements at 100,000 cells per ml. A total of 300,000 cells per animal were injected into six-week-old athymic mice using the Stoelting stereotactic injection apparatus and a sharp Hamilton syringe. Mice were anaesthetized with isofluorane and placed in the stereotactic frame using ear bars and constant isofluorane supply through a mouthpiece adaptor. A hole was bored in the skull 1 mm anterior and 0.5 mm lateral to the Bregma, and 2.5 mm below the surface of the brain and cells were injected using manual pressure. Mice were followed by bioluminescence imaging until luminescence signal indicated that tumours were established. Radiation was administered at 4 Gy using the JLShepherd @ Associates irradiator (model: MK1-68) three times per week, followed by bioluminescence imaging one day after each treatment. On day 13 after treatment start, mice were killed, perfused with 4% paraformaldehyde, brains were isolated and fixed overnight in 4% paraformaldehyde, then transferred to 70% ethanol for processing. Mouse brain specimens were serially sectioned and paraffin embedded using standard methods. Haematoxylin and eosin sections were prepared by routine methods. Antigen retrieval for immunohistochemistry was performed in Tris-EDTA, pH 8.0, for 30 min at 95 °C. Slides were treated with blocking reagent (Vector M.O.M. kit BMK-2202) for 32 min. Immunohistochemistry was performed using primary antibodies for Ki67 (Ventana RRF 790–4286, undiluted, room temperature for 16 min) or cleaved caspase 3 (Cell Signaling, #9661, diluted 1:50 in M.O.M. diluent, 37 °C for 60 min). Antibody detection was performed using the Ventana IView Detection Kit (760-091). How to cite this article : Bakhoum, S. F. et al . Numerical chromosomal instability mediates susceptibility to radiation treatment. Nat. Commun. 6:5990 doi: 10.1038/ncomms6990 (2015).